Identification of four novel susceptibility loci for oestrogen receptor negative breast cancer Common variants in 94 loci have been associated with breast cancer including 15 loci with genome-wide significant associations ( P <5 × 10 −8 ) with oestrogen receptor (ER)-negative breast cancer and BRCA1 -associated breast cancer risk. In this study, to identify new ER-negative susceptibility loci, we performed a meta-analysis of 11 genome-wide association studies (GWAS) consisting of 4,939 ER-negative cases and 14,352 controls, combined with 7,333 ER-negative cases and 42,468 controls and 15,252 BRCA1 mutation carriers genotyped on the iCOGS array. We identify four previously unidentified loci including two loci at 13q22 near KLF5 , a 2p23.2 locus near WDR43 and a 2q33 locus near PPIL3 that display genome-wide significant associations with ER-negative breast cancer. In addition, 19 known breast cancer risk loci have genome-wide significant associations and 40 had moderate associations ( P <0.05) with ER-negative disease. Using functional and eQTL studies we implicate TRMT61B and WDR43 at 2p23.2 and PPIL3 at 2q33 in ER-negative breast cancer aetiology. All ER-negative loci combined account for ∼ 11% of familial relative risk for ER-negative disease and may contribute to improved ER-negative and BRCA1 breast cancer risk prediction. Breast cancer is a heterogeneous disease that can be separated into clinical subtypes based on tumour histological markers, such as the oestrogen receptor (ER). ER-negative disease accounts for 20–30% of all breast cancers, is more common in women diagnosed at young age and in women of African ancestry [1] , and is associated with worse short-term outcome than ER-positive disease. ER-negative and ER-positive breast cancer also exhibit different patterns of genetic susceptibility [2] . Currently, 94 loci containing common breast cancer risk-associated variants have been associated with breast cancer through genome-wide association studies (GWAS), and large replication studies [3] , [4] , [5] , [6] , [7] , [8] , [9] , [10] , [11] , [12] , [13] , [14] , [15] , [16] , [17] , [18] . However, only 14 loci have shown genome-wide significant associations ( P <5 × 10 −8 ) with ER-negative disease [3] , [17] , [18] , [19] , [20] . While this partly reflects the smaller sample size for ER-negative disease, the majority of the known breast cancer loci show differences in relative risk by subtype. In particular, 6 of the 14 loci associated with ER-negative disease at genome-wide significance show no evidence of association with ER-positive disease [20] . The alleles associated with ER-negative breast cancer [3] , [17] at these loci have also been associated with breast cancer risk in BRCA1 mutation carriers [21] , [22] , consistent with the finding that the majority of breast tumours arising in BRCA1 mutation carriers show low/absent expression of ER [23] , [24] , [25] . These observations suggest that a meta-analysis of results from ER-negative breast cancer and BRCA1 breast cancer association studies could identify additional ER-negative susceptibility loci that were not found previously because of limited sample size. In this study, we carried out a meta-analysis of breast cancer GWAS studies and found four new loci associated with developing ER-negative breast cancer. 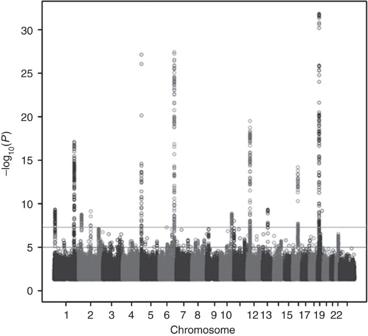Figure 1: Manhattan plot of ER-negative breast cancer meta-analysis. The Manhattan plot displays the strength of genetic association (−log10P) versus chromosomal position (Mb), where each dot presents a genotyped or imputed (black circle) SNP. The black horizontal line represents the threshold for genome-wide significance (P=5 × 10−8). Associations with ER-negative breast cancer Genotype data for this meta-analysis were obtained from three sources: (1) 11 breast cancer GWAS included 5,139 ER-negative breast cancer cases and 14,352 controls ( Supplementary Table 1 ); (2) The Breast Cancer Association Consortium (BCAC) included 7,333 ER-negative breast cancer cases and 42,468 study-matched controls genotyped on the iCOGS (Collaborative Oncological Gene-environment Study) custom array [3] ; (3) The Consortium of Investigators of Modifiers of BRCA1/2 (CIMBA) [26] included 15,252 BRCA1 mutation carriers (7,797 with breast cancer and 7,455 unaffected) genotyped on the iCOGS array ( Supplementary Tables 2–4 ). Imputation was performed using the 1000 Genomes project as a reference [20] , [27] , and a meta-analysis was performed based on 10,909,381 common single-nucleotide polymorphisms (SNPs) that passed quality control ( Supplementary Table 1 ). We first considered SNPs in 94 regions in which genome-wide significant associations for breast cancer had been identified (Methods) [20] . In 55 of these, the SNP most significantly associated with overall breast cancer risk was significantly associated ( P <0.05) with ER-negative breast cancer in the meta-analysis. Four more were associated with ER-negative breast cancer in the general population ( P <0.05) but not in the meta-analysis, and 15 displayed genome-wide significant ( P <5 × 10 −8 ) associations with ER-negative breast cancer ( Supplementary Table 5 ). In addition, new SNPs in three loci (rs10864459 from 1p36.2 PEX14 , rs11903787 from INHBB and rs4980383 from 11p15.5 LSP1 ) were found to have genome-wide significant associations with ER-negative disease ( Table 1 , Fig. 1 , Supplementary Table 5 ). Likewise, SNPs in the TCF7L2 locus previously associated with BRCA1 breast cancer [22] and ER-positive breast cancer [3] , [20] showed genome-wide significant associations with ER-negative breast cancer ( Table 1 ). Interestingly multiple independent signals in several loci were associated with ER-negative breast cancer. In particular, three independent regions in the TERT locus [28] , two regions in PTHLH, and two regions in ESR1 displayed genome-wide significant associations with ER-negative breast cancer ( Table 1 ). Furthermore, while previous studies established genome-wide significant associations with ER-negative disease for rs11075995 in one 16q12.2 FTO locus [17] , rs17817449 ( r 2 =0.035) from a second FTO locus located 40 kb proximal to the rs11075995 tagged locus [17] also displayed near-genome-wide significance ( P =5.26 × 10 −8 ) with ER-negative breast cancer in the meta-analysis ( Table 1 ). In addition to the breast cancer loci established in studies of European women, three additional breast cancer risk loci were recently identified in GWAS of Asian women. To generalize the results to other populations, associations between the three SNPs and breast cancer in the European, African American and Asian populations in the iCOGS study were evaluated. SNP rs2290203 showed only weak evidence of association ( P =0.02), and rs4951011 and rs10474352 SNPs showed no evidence of association with ER-negative breast cancer in the white European meta-analysis ( Supplementary Table 6 ). Table 1 Common genetic variants from known breast cancer susceptibility loci displaying most significant genome-wide associations with ER-negative breast cancer risk. Full size table Figure 1: Manhattan plot of ER-negative breast cancer meta-analysis. The Manhattan plot displays the strength of genetic association (−log 10 P ) versus chromosomal position (Mb), where each dot presents a genotyped or imputed (black circle) SNP. The black horizontal line represents the threshold for genome-wide significance ( P =5 × 10 −8 ). Full size image Among the 94 known risk loci from white European and three from Asian populations, only 24 contained SNPs with some evidence of association ( P <0.05) with breast cancer risk among BRCA1 mutation carriers alone. These included 21 loci based on known index SNPs ( Supplementary Table 5 ) along with new SNPs from the meta-analysis in the PEX14 (rs10864459), INHBB (rs11903787) and PTHLH (rs7297051) loci ( Table 1 ). Only the ESR1 (rs2046210), TERT (rs2242652) and two 19p13.1 (rs8170; rs56069439) loci had genome-wide significant associations with breast cancer risk for BRCA1 mutation carriers alone ( Table 1 , Supplementary Table 5 ). However, 15 of the 19 risk loci that reached genome-wide significance for ER-negative disease in the meta-analysis showed some evidence of association ( P <0.05) with breast cancer risk for BRCA1 mutation carriers using a retrospective likelihood analysis [12] . These SNPs had hazard ratio (HR) estimates in BRCA1 carriers that were similar to the odds ratio (OR) estimates for ER-negative breast cancer ( Table 1 ). In contrast, four SNPs in the LGR6 , 2p24.1 , ZNF365 and FTO loci had HR estimates ranging from 0.97 to 1.01 and were not significantly associated ( P >0.05) with breast cancer risk for BRCA1 mutation carriers. No significant interactions between the known risk SNPs were observed when pairwise interactions were evaluated separately in the general population (BCAC-iCOGS) or in BRCA1 carriers after adjusting for multiple testing. 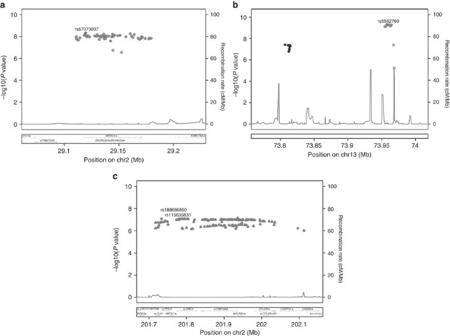Figure 2: Novel ER-negative breast cancer loci. The chromosomal position and strength of genetic association (−log10P) is shown for all SNPs (P<1 × 10−6) in BCAC/iCOGS data in the four novel risk loci. (a). 2p23 locus. The most significant SNP (rs67073037) is shown as a diamond. (b). 13q22 loci. The most significant SNP (rs6562760) is shown as a diamond. The second locus is shown in black. (c). 2q33 locus. The most significant SNPs (rs188686860; rs115635831) are shown as diamonds. Genome-wide associations with ER-negative breast cancer Novel genome-wide significant associations ( P <5 × 10 −8 ) were detected with imputed and genotyped SNPs on chromosomes 2p23.2 and 13q22 ( Table 2 , Fig. 2 , Supplementary Fig. 1 ). At 2p23.2, 79 SNPs exhibited genome-wide significant associations with ER-negative breast cancer ( Fig. 2 , Supplementary Fig. 2 , Supplementary Table 7 ). The most significant genotyped and imputed SNPs at these two loci were rs4577244 ( P =1.0 × 10 −8 ) and rs67073037 ( P =4.76 × 10 −9 ), respectively ( Table 2 ). To investigate the presence of independent signals at the 2p23.2 locus, conditional analyses were conducted adjusting for the lead SNP. However, no significant ( P <0.05) associations were observed at 2p23.2 after adjusting for rs67073037. In the 13q22 locus, rs6562760 was the most strongly associated ( P =5.0 × 10 −10 ) SNP among 12 genome-wide significant SNPs ( Table 2 , Supplementary Table 8 , Fig. 2 , Supplementary Fig. 1 ). Conditional analysis adjusting for rs6562760 yielded several SNPs with residual associations for ER-negative breast cancer, with rs17181761 ( r 2 =0.51) as the most significantly associated ( P =6.0 × 10 −6 ) ( Supplementary Table 9 ). No associations at P <10 −4 remained after conditioning on both rs6562760 and rs17181761. Thus, 13q22 appears to contain two independent ER-negative risk loci. Table 2 Novel associations of common genetic variants with ER-negative breast cancer risk. Full size table Figure 2: Novel ER-negative breast cancer loci. The chromosomal position and strength of genetic association (−log 10 P ) is shown for all SNPs ( P <1 × 10 −6 ) in BCAC/iCOGS data in the four novel risk loci. ( a ). 2p23 locus. The most significant SNP (rs67073037) is shown as a diamond. ( b ). 13q22 loci. The most significant SNP (rs6562760) is shown as a diamond. The second locus is shown in black. ( c ). 2q33 locus. The most significant SNPs (rs188686860; rs115635831) are shown as diamonds. Full size image When considering only the data from the general population using the BCAC-iCOGS studies, no association between rs67073037 at 2p23.2 and ER-positive breast cancer was observed ( Supplementary Table 10 ). Consistent with this observation, a significant difference ( P diff =4.45 × 10 −6 ) in the per-allele ORs for ER-positive and ER-negative breast cancer was detected. In contrast, rs17181761 at 13q22 was weakly associated with ER-positive breast cancer (OR=1.03; P =0.030), but more strongly associated with ER-negative breast cancer (OR=1.08; P diff =5.82 × 10 −3 ; Supplementary Table 10 ). Likewise, rs6562760 at 13q22 was more strongly associated with ER-negative than ER-positive breast cancer (ER-positive OR=0.98 versus ER-negative OR=0.92; P diff =0.028) ( Supplementary Table 10 ). Among ER-negative cases, no significant differences in the ORs for triple negative (ER-negative, progesterone receptor negative, HER2 negative) and non-triple-negative cases was observed (rs67073037, P diff =0.26; rs6562760, P diff =0.36; rs17181761, P diff =0.69). Q-tests were used to assess heterogeneity. These results suggest that the three risk loci are largely specific to ER-negative but not triple-negative breast cancer, in contrast to loci in the MDM4 , LGR6 , 19p13.1 and TERT regions [3] , [17] . To also investigate the impact of bilateral disease on the associations with ER-negative breast cancer in the general population, analyses were performed separately for BBCS alone, which oversampled for bilateral cases, and after exclusion of BBCS. The risk estimates for each SNP (both in iCOGS and in the meta-analysis), after excluding BBCS, did not differ from the main results ( Supplementary Table 11 ), and do not appear to be substantially influenced by bilateral cases. Using the retrospective likelihood approach, index SNPs in the three 2p23.2 and 13q22 loci were all associated with BRCA1 breast cancer (rs67073037, P =4.58 × 10 −4 ; rs6562760, P =2.85 × 10 −6 ; rs17181761, P =9.29 × 10 −3 ; Table 2 ). There were no significant differences in the associations with ER-positive and ER-negative disease among BRCA1 carriers ( Supplementary Table 12 ). A competing risks analysis in BRCA1 mutation carriers that accounted for simultaneous associations with breast and ovarian cancer risks found similar HR estimates for breast cancer and no evidence of association with ovarian cancer risk ( Supplementary Table 13 ). None of the SNPs were associated with overall breast cancer risk for BRCA2 mutation carriers ( Supplementary Table 10 ). There was also no significant evidence of heterogeneity ( P <0.05) between the effect estimates for BRCA1 mutation carriers and ER-negative breast cancer in the general population (BCAC-iCOGS; Intraclass Correlation) [27] . Finally, no significant interactions between the three index SNPs and any of the 94 previously known loci were observed in BRCA1 carriers or in the general population after adjusting for multiple testing ( Supplementary Table 14 ). Association with ER-negative breast cancer in the 2q33 locus Analysis of genotyped and imputed SNPs around known risk loci also detected near-genome-wide significant associations with ER-negative breast cancer in a region on 2q33 containing several genes including PPIL3 and the known CASP8 risk locus ( Table 2 ). rs115635831 ( P =1.26 × 10 −7 ) and rs188686860 ( P =8.34 × 10 −8 ; r 2 =1.0), were the genotyped and imputed SNPs, respectively, most significantly associated with ER-negative breast cancer in this region. These SNPs, along with the most proximal rs74943274 SNP ( r 2 =0.97 with rs115635831), are located in CLK1 (Cdc-like kinase-1) and PPIL3 (Peptidylproplyl isomerase-Like 3) and are 350 kb upstream of CASP8 ( Table 2 , Fig. 2 ). All 157 SNPs with highly significant associations ( P <1 × 10 −6 ) in this region, were in high linkage disequilibrium with rs188686860 and rs115635831 ( r 2 >0.90), and were located proximal (Hg19: 201,717,014-201,995,860) to the CASP8 gene ( Supplementary Table 15 ). Fine mapping of the CASP8 locus has recently identified four independent signals associated with overall breast cancer risk [29] . The index SNPs for these independent signals range across a 350-kb region from 202,036,478 to 202,379,828. To determine whether these CASP8 -associated signals accounted for the ER-negative associations in the meta-analysis, conditional analyses were conducted using the BCAC-iCOGS data. After accounting for the four CASP8 signals, rs74943274 retained evidence of an association with overall breast cancer ( P =1.44 × 10 −3 ) and a strong association with ER-negative breast cancer ( P =1.34 × 10 −5 ; Supplementary Table 16 ; Supplementary Fig. 2 ), suggesting that rs74943274 and rs115635831 represents a novel locus associated with ER-negative breast cancer. Further consideration of the BCAC-iCOGS data found no association for rs115635831 at 2q33 with ER-positive breast cancer ( P =0.23) but identified a significant difference ( P diff =2.9 × 10 −4 ) in the per-allele ORs for ER-positive and ER-negative breast cancer (Q-test, Supplementary Table 10 ). No influence of bilateral disease was observed in sensitivity analyses ( Supplementary Table 11 ). However, the index SNPs in the 2q33 locus were significantly associated with BRCA1 breast cancer (rs115635831, P =0.018; rs188686860, P =0.012; Table 2 ). While there were no significant differences in the associations with ER-positive and ER-negative disease among BRCA1 carriers ( P Het=0.12), the associations were stronger for ER-negative (rs115635831 HR=1.32, P =3 × 10 −3 ) than ER-positive breast cancer (rs115635831 overall HR=1.21, P =0.018) using the retrospective likelihood model ( Supplementary Table 12 ). In addition, the associations for BRCA1 mutation carriers were of similar magnitude as the OR estimates for ER-negative breast cancer in BCAC-iCOGS [27] ( Supplementary Table 15 ). There was also no evidence of intraclass heterogeneity ( P <0.05) between the effect estimates for BRCA1 mutation carriers and ER-negative breast cancer in the general population (BCAC-iCOGS) [27] . A competing risks analysis for BRCA1 mutation carriers found little influence of ovarian cancer on risks of breast cancer (rs115635831 HR=1.23, P =0.016), and no evidence of association with ovarian cancer risk using the retrospective likelihood model ( Supplementary Table 13 ). No association with overall breast cancer risk among BRCA2 mutation carriers ( Supplementary Table 10 ) was evident. Interestingly, rs114962751 at 2q33 and rs150750171 at 6p had the most significant interaction ( P =3.9 × 10 −4 ) among all known breast cancer risk SNPs in the iCOGS data, although the interaction was non-significant after adjusting for multiple testing ( Supplementary Table 14 ). Altogether these results suggest the presence of a novel locus associated with ER-negative breast cancer that is located in the CLK1/PPIL3 region proximal to CASP8 . Expression quantitative trait locus (eQTL) analysis To identify the genes in the novel loci influenced by the observed associations with ER-negative breast cancer, expression quantitative trait locus (eQTL) analyses were performed using gene expression data from breast tumour tissue and normal breast tissue and 1000 Genomes Project imputed SNPs in 1 Mb regions around the novel loci. In the 2p23.2 locus, the strongest cis eQTL associations for 735 TCGA breast tumours (BC765) involved TRMT61B expression ( Supplementary Table 17 ). Most of the genome-wide significant ER-negative breast cancer risk SNPs in the locus displayed associations with TRMT61B expression, including the imputed SNPs (rs67073037, P =1.47 × 10 −5 ; Supplementary Fig. 3 ; rs6734079, P =1.85 × 10 −5 ) and the genotyped SNP (rs4577254, P =5.61 × 10 −5 ) most significantly associated with risk ( Supplementary Table 18 ). Similarly, in a Norwegian normal breast cohort of 116 normal breast tissues (NB116), the strongest cis eQTLs associations involved TRMT61B expression and the risk SNPs in the locus yielded significant associations with TRMT61B expression ( Supplementary Table 17 ). While the peak eQTL SNPs (rs6419696, P =1.21 × 10 −17 ) were not among the SNPs showing the greatest association with risk (rs6419696, P =2.6 × 10 −3 ), conditional analyses showed that the rs6419696 eQTL SNP accounted for much of the influence of the rs4577254 SNP on ER-negative breast cancer risk ( P =9.07 × 10 −4 ) and vice versa ( Supplementary Table 18 ). Thus, modulation of TRMT61B expression may contribute in part to the risk of breast cancer in this region. In the 13q22.1 locus, the strongest eQTLs in the 735 TCGA breast tumours (BC765) involved PIBF1 ( Supplementary Table 19 ). However, none of the SNPs strongly associated with breast cancer risk in either of the two independent 13q22 loci showed associations with gene expression ( Supplementary Table 19 , Supplementary Fig. 4 ). In contrast, significant associations with DIS3 expression were observed in the BC241 and NB116 cohorts for many of the genome-wide significant SNPs in the locus represented by rs17181761 (NB116 eQTL P =2.34 × 10 −3 ) ( Supplementary Table 19 ). While non-significant after accounting for multiple testing, these observations suggest that future studies should evaluate mechanistic interactions between 13q22.1 SNPs and DIS3 expression. Evaluation of eQTLs in the 2q33 locus for the BC765 cohort found that many of the 157 risk-associated SNPs ( Table 2 , Supplementary Table 15 ) had strong associations with PPIL3 expression (rs188686860, P =1.77 × 10 −7 ; rs115635831, P =6.08 × 10 −7 ; Supplementary Fig. 5 ) and little evidence of any associations with other genes in the region ( Supplementary Table 20 ). This is one of the few known breast cancer risk loci where the most significant risk SNPs are strongly associated with local gene expression. PPIL3 is located at the proximal end of the locus, 270 kb upstream of CASP8 , further suggesting that the 2q33 risk locus is independent of any influence on CASP8 . Functional characterization of the 2p23.2 locus To identify candidate SNPs and genes in the 2p23.2 locus driving ER-negative breast cancer risk, ENCODE chromatin biofeatures were evaluated in primary human mammary epithelial cells (HMECs), MCF7 ER-positive cells and MB-MDA-231 ER-negative cells [30] . Sixteen of the 79 most significantly associated SNPs ( P <3 × 10 −7 ) in the region overlapped with three distinct regulatory regions ( Supplementary Figs 6 and 7 ). The most significantly associated ER-negative SNP, rs67073037 ( Table 2 ) was located in intron 1 of WDR43 near the transcription start site in a region containing acetylated H3K27 and trimethylated H3K4 chromatin marks in normal HMECs and MB-MDA-231 ER-negative breast tumour cells, and a DNase hypersensitivity cluster in ER-positive MCF7 cells ( Supplementary Figs 6 and 7 ). The three risk-associated SNPs (rs4407214, rs66604446 and rs66768547) with the most significant RegulomeDB scores (2b), were located in the same chromatin marks in this region in HMEC, MD-MBA-231 and MCF7 cells ( http://regulomedb.org ). In addition, the top genotyped SNP (rs4577244) was located in a monomethylated H3K4 mark adjacent to the core promoter region of WDR43 in HMECs ( Supplementary Fig. 6 ). Separately rs11677283 and rs35617956 in introns 9 and 10 of WDR43 were located in acetylated H3K27 and H3K9 chromatin marks in a putative regulatory region in HMECs, but not in ER-negative MD-MBA-231 cells. Combining the eQTL results with these predictions, we tested four genomic tiles spanning region 1 for enhancer activity in both orientations using a luciferase reporter assay in the CAL51 ER-negative breast cancer line and MCF10A normal mammary epithelial cells ( Fig. 3 ). The tile containing rs4407214 displayed significant enhancer activity ( P <0.0001) in at least one orientation when compared with the negative control in MCF10A and CAL51 ( Fig. 3 ). In addition, the tile carrying the disease-associated G allele showed significantly ( P =0.0059) higher activity than the T allele in MCF10A cells ( Fig. 3 ). Similarly, the disease-associated G-allele showed significantly ( P =0.0059) higher activity than the T-allele in a luciferase-based promoter assay in MCF10A cells ( P =0.044) and CAL51 ( P =0.0078; Supplementary Fig. 8 ). Consistent with these allele-specific changes in transcriptional activity different protein complexes in electrophoretic mobility shift assays were observed using CAL51 and MCF10A nuclear extracts ( Fig. 3 ). In addition, Pol2 ChIA-PET in MCF7 breast cancer cells revealed an interaction between Region 1 and the promoter of TRMT61B ( Fig. 3 ), which had the strongest eQTL signal in the locus. These results are consistent with modification of Pol2 binding to this region by rs4407214 in lymphoblastoid cells [31] and suggest the presence of a transcriptional enhancer in the region. Separately, the ChIA-PET data further suggest that Region 2 in WDR43 may interact with the promoter of WDR43 ( Fig. 3 ). Thus, WDR43 and TRMT61B may be regulated by interactions of enhancers in WDR43 with the core WDR43 and TRMT61B promoters and may jointly influence breast cancer risk in this region. 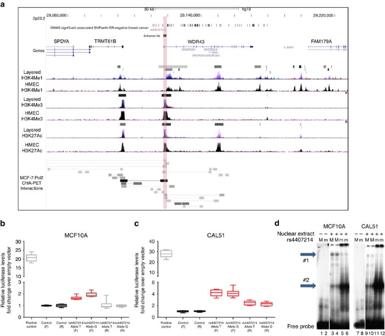Figure 3: The chromatin landscape of locus 2p23.2. (a) The SNP rs4407214 is included in a genomic tile overlapping chromatin features indicative of promoters and enhancers, shaded red. (b,c). Luciferase assays showing activity in the tile containing SNP rs4407214 (highlighted in pink ina.) in MCF10A and CAL51, red box plots indicate significantly different from the control tile (P<0.0001). Brown box plot indicates significant difference from the reference allele (P= 0.0059). (d) Electrophoretic mobility shift assay (EMSA) showing the formation of allele-specific complexes for rs4407214. M, major allele; m, minor allele. Lines 1, 2, 7, 8—no nuclear extract. Lines 3, 4, 5, 6—10 μg of MCF10A nuclear extract. Lines 9, 10, 11, 12—10 μg of CAL51 nuclear extract. Shift detected by comparison to bands (arrows #1 and #2). Figure 3: The chromatin landscape of locus 2p23.2. ( a ) The SNP rs4407214 is included in a genomic tile overlapping chromatin features indicative of promoters and enhancers, shaded red. ( b , c ). Luciferase assays showing activity in the tile containing SNP rs4407214 (highlighted in pink in a .) in MCF10A and CAL51, red box plots indicate significantly different from the control tile ( P <0.0001). Brown box plot indicates significant difference from the reference allele ( P = 0.0059). ( d ) Electrophoretic mobility shift assay (EMSA) showing the formation of allele-specific complexes for rs4407214. M, major allele; m, minor allele. Lines 1, 2, 7, 8—no nuclear extract. Lines 3, 4, 5, 6—10 μg of MCF10A nuclear extract. Lines 9, 10, 11, 12—10 μg of CAL51 nuclear extract. Shift detected by comparison to bands (arrows #1 and #2). Full size image Functional characterization of the 13q22 locus The SNPs most significantly associated with ER-negative breast cancer in the two 13q22 loci formed two small clusters in a 4-kb region around rs17181761 and a 10-kb region around rs8002929. Bioinformatics analysis and chromatin feature analysis identified weak DNaseI hypersensitivity sites, CTCF binding and monomethylated H3K4 sites in both regions in HMEC cells, consistent with weak enhancer activity ( Supplementary Figs 9 and 10 ). Both rs17181761 and rs12870942 in the proximal locus are associated with transcriptional activity in HMECs, whereas rs8002929 and rs927683 in the distal locus are associated with enhancer and DNAse hypersensitivity sites in HMECs, respectively ( http://regulomedb.org ). Both 13q22 loci are located in a non-genic 600-kb region between the KLF5 and KLF12 kruppel-like transcription factor genes. This segment of chromosome 13 is frequently deleted in a spectrum of cancers [32] , [33] . GWAS have also identified a pancreatic cancer risk locus in the region between KLF5 and KLF12 (refs 34 , 35 , 36 ). However, the rs9543325 SNP from the pancreatic cancer studies was only marginally associated with ER-negative breast cancer risk ( P =0.03) in the meta-analysis suggesting that the signals are independent. Functional characterization of the 2q33 locus The SNPs most significantly associated with ER-negative breast cancer in the 2q33 locus range across a 350-kb region that contains nine genes ( Supplementary Fig. 6 ). This region contains at least 10 strong enhancer regions in HMECs and 12 strong enhancer regions in MD-MBA-231 cells associated with acetylated H3K27 and trimethylated H3K4 chromatin marks. As noted above, many of the 157 SNPs most significantly associated with ER-negative breast cancer are associated with PPIL3 expression. Seven of these also scored as functional candidates by RegulomeDB (score=3a; rs17467658, rs17383256, rs17467916, rs114567273, rs76377168, rs116509920 and rs116724456). Of these rs17467658 in CLK1 and rs17383256 in the ORC2 gene are located in DNAse hypersensitivity sites and strong enhancer regions in HMEC and MD-MBA-231 cells ( http://www.roadmapepigenomics.org ; Supplementary Figs 11 and 12 ). In addition, rs116509920 and rs116724456 are associated with PPIL3 expression ( P =5.85 × 10 −7 ), although neither SNP is associated with an enhancer or suppressor region. The genotyped SNP most significantly associated with risk, rs114962751, is located in acetylated H3K27 and trimethylated H3K4 chromatin marks in a bidirectional promoter for FAM126B and NDUFB3 in HMEC and MD-MBA-231 cells ( Supplementary Figs 11 and 12 ). Similarly, the rs74943274 genotyped risk SNP ( Table 2 ) is located near the 3′-untranslated region of CLK1 and is associated with PPIL3 expression ( P =2.37 × 10 −6 ). However, rs78258606 is perhaps a more likely candidate driver of ER-negative risk in this locus because the SNP is associated with ER-negative breast cancer ( P =1.9 × 10 −7 ), is located in the CLK1 promoter in acetylated H3K27 and trimethylated H3K4 chromatin marks in HMEC and MD-MBA-231 cells and DNase hypersensitivity sites in MCF7 cells, and is associated with PPIL3 expression ( P =2.71 × 10 −7 ) ( Supplementary Figs 11 and 12 ). Further fine mapping and functional characterization of this locus is needed to resolve the underlying functional effects and identify the genes influencing ER-negative breast cancer risk. When including the four 2p23.2, 13q22 and 2q33 novel loci identified in this meta-analysis, 23 independent loci have shown genome-wide significant associations with ER-negative disease, including 10 loci showing no associations or only weak associations with ER-positive disease. In total, 63 loci have shown at least marginal significance ( P <0.05) with ER-negative breast cancer. In BRCA1 mutation carriers, 27 independent loci ( P <0.05) have been associated with modified breast cancer risk [27] . The percentage of the familial risk for ER-negative disease explained by SNPs is not well defined because there is currently no good estimate for the familial relative risk for ER-negative disease. However, assuming that the estimate is similar to that for overall breast cancer (twofold for a first-degree relative), and based on the estimated frequencies and ORs from the iCOGS data, the SNPs in the known breast cancer risk loci explain 9.8% of the familial risk and the SNPs in the four new loci account for a further 0.8%. The addition of these new ER-negative loci may improve overall risk prediction models for ER-negative disease in the general population and for breast cancer among BRCA1 mutation carriers by enhancing the contribution of current polygenic risk prediction models [21] , [22] . Furthermore, fine mapping and functional studies of these loci may provide further insight into the aetiology of ER-negative breast cancer. Study populations Details of the subjects, genotyping and quality control measures for the BCAC GWAS and iCOGS data [3] , BPC3 (ref. 16 ), EBCG [37] , TNBCC [14] , [38] and BRCA1 (ref. 22 ) are described elsewhere. Analyses were restricted to women of European ancestry. Overall, 42 BCAC studies provided the iCOGS genotyping data for ER-negative breast cancer cases and controls. In addition, 11 breast cancer studies provided GWAS genotyping data. Forty five CIMBA studies provided iCOGS genotyping on 15,252 BRCA1 mutation carriers, of whom 7,797 were affected with breast cancer. Genotype data Genotyping and imputation details for each study are shown in Supplementary Table 1 . Imputation We performed imputation separately for BRCA1 carriers, 11 GWAS, BCAC-iCOGS and TNBCC-iCOGS samples. We imputed variants from the 1000 Genomes Project data using the v3 April 2012 release [39] as the reference panel. Imputation was based on the 1000 Genomes Project data with singletons removed. Eight BCAC GWAS were imputed in a two-step procedure, with prephasing using the SHAPEIT software and imputation of the phased data in the second with IMPUTEv2 (ref. 40 ). For the remaining three GWAS (BPC3, TNBCC and EBCG), imputation was performed using MACH (version 1.0.18) and Minimac (version 2012.8.15) [41] . The iCOGS data were also imputed with two-stage procedure involving SHAPEIT and IMPUTEv2. To perform the imputation we divided the data into segments of ∼ 5 Mb each. The iCOGS samples were divided into 10 subsets, keeping all subjects from individual studies in the same set. Estimates and s.e.’s were obtained using logistic regression adjusting for study and 9 principal components. GWAS SNPs were excluded if the imputation accuracy was r 2 <0.3 or if the minor allele frequency (MAF) was <0.01, TNBCC SNPs were excluded when the imputation accuracy was r 2 <0.9 and MAF<0.05, iCOGS SNPs were excluded when r 2 <=0.3 and MAF<0.005. Regions with evidence of genome-wide significant associations ( P <5 × 10 −8 ) were reimputed in iCOGS, using IMPUTEv2 but without prephasing in SHAPEIT to improve imputation accuracy. In addition, the number of MCMC iterations were increased from 30 to 90, and the buffer region was increased to ±500 kb from any significantly associated SNP in the region. Meta-analysis A fixed effects meta-analysis of ER-negative breast cancer associations was conducted using an inverse variance approach assuming fixed effects, as implemented in METAL [42] . The effect estimates used were the logarithm of the per-allele HR estimate for the association with breast cancer risk in BRCA1 and BRCA2 mutation carriers and the logarithm of the per-allele OR estimate for the association with breast cancer status in GWAS and iCOGS analyses, both of which were assumed to approximate the same relative risk. For the associations in BRCA1 mutation carriers, a kinship-adjusted variance estimator was used [12] . P -values were estimated by z -test. Heterogeneity analysis Heterogeneity across estimates from BCAC and iCOGS were evaluated using a Cochran Q test and I 2 for the proportion of total variability explained by heterogeneity in the effect sizes [43] . Associations with ER-positive and ER-negative subgroups of BRCA1 carriers were evaluated using an extension of the retrospective likelihood approach to model the simultaneous effect of each SNP on more than one tumour subtype [27] . The consistency between breast cancer associations for breast cancer susceptibility variants in the general population and associations in BRCA1 and BRCA2 carriers were evaluated using the intraclass correlation (ICC) [27] . The ICC was estimated based on a one-way random-effects model and tested for agreement in absolute values of log HR. Locus coverage Locus boundaries were defined so that all SNPs with r 2 ⩾ 0.1 with the most significantly associated SNP were included. SNPs with MAF<0.005 were excluded. Linkage disequilibrium blocks were defined at r 2 ⩾ 0.8. Each linkage disequilibrium block was evaluated for the presence of at least one genotyped or imputed SNP. If imputed, then the imputation accuracy was considered. Expression quantitative trait locus analysis eQTL analysis was performed for all protein coding genes within 1 Mb, up- and downstream of the SNP most significantly associated with ER-negative breast cancer risk in each locus. Normal breast (NB116; n =116) and breast cancer (BC241, n =241) are comprised of women of Norwegian descent. Gene expression data for the majority of women in NB116 were derived from normal breast tissue in women who had not been affected with breast cancer; data for ten women were derived from normal tissue adjacent to a tumour. Gene expression data for BC241 were derived from breast tumours (70 ER-negative and 170 ER-positive). Genotyping was performed with the iCOGS SNP array, and gene expression levels were measured with the Agilent 44K array [44] , [45] . BC765 ( n =765) is the TCGA breast cancer cohort composed of 139 ER-negative, 571 ER-positive and 55 undefined breast tumours; all non-European samples (as determined by clustering and PCA) were excluded from this analysis [46] . Germline genotype data from Affymetrix SNP 6 array were obtained from TCGA dbGAP data portal [46] . Gene expression levels for the breast tumours were assayed by RNA sequencing, RSEM (RNaseq by Expectation-Maximization21) normalized per gene, as obtained from the TCGA consortium portal [46] . The data were log2 transformed, and unexpressed genes were excluded prior to eQTL analysis. There is no overlap between women recruited to each of these studies. The genotyping data were processed as follows: SNPs with call rates <0.95 or minor allele frequencies <0.05 or Hardy–Weinberg equilibrium ( P <10 −13 ) were excluded. Samples with call rates below 80% were excluded. Identity by state was computed with the R GenABEL package [47] and closely related samples with IBS>0.95 were removed. Imputation was performed on the iCOGS and Affymetrix6 germline genotype data using the 1000 Genomes Project March 2012 v.3 release as the reference data set. A two-stage imputation procedure was used as described above. The influence of SNPs on gene expression was assessed using a linear regression model. An additive effect was assumed by modelling copy number of the rare allele, that is, 0, 1 or 2, for a given genotype. Candidate gene analysis TCGA has performed extensive genomic analysis of tumours from a large number of tissue types including over 1,000 breast tumours. All genes in the novel loci were evaluated for coding somatic sequence variants in TCGA. Breast tumours with log2 copy-number data in the TCGA data were analysed for deletion and amplification of each candidate gene using the cBio portal [48] , [49] . Informatics and chromatin biofeatures Candidate SNPs were evaluated using SNPInfo ( http://snpinfo.niehs.nih.gov ) and SNPnexus ( http://snp-nexus.org/test/snpnexus ). The presence of SNPs in transcription factor binding sites using TRANSFAC and miRNA binding sites using TargetScan were noted. Regulatory potential scores (ESPERR Regulatory Potential) were obtained from the UCSC genome bioinformatics browser ( http://genome.ucsc.edu/ ). RegulomeDB ( http://regulomedb.org ) was used to assess SNPs for transcription factor recognition motifs, open chromatin structure based on FAIRE and DNAse-seq analysis and protein binding sites based on ChIP-seq data. Chromatin biofeatures in HMEC and MCF7 cells were assessed using ENCODE layers on the UCSC browser ( http://genome.ucsc.edu/ ). Enhancers active in the mammary cell types MCF7 and HMEC were cross-referenced with candidate SNPs. Luciferase reporter assays Genomic tiles spanning regions containing SNPs with indication of regulatory activity by RegulomeDB were generated. Regions containing the major and minor alleles within the 2p23.2 region spanning 2,229 bp (chr2:29,117,333-29,119,561) were generated by PCR using BAC DNA CTD-3216P10 as template. Forward and reverse primers contained att B1 and att B2 sequences, respectively, to aid in recombinational cloning. Tiles were cloned in both a forward and reverse orientation upstream of the SV40 promoter by recombination in the firefly luciferase reporter vector pGL3-Pro-attb vector designed to test for enhancer regions. This vector is a modification of pGL3-Promoter (Invitrogen) adding att B sites surrounding the ccdb gene. The clone containing the tile was co-transfected in eight replicates using LipoFectamine 2000 (Life Technologies) into MCF10A or CAL51 cells with pRL-CMV (Promega), an internal control expressing Renilla luciferase, per well of 96-well plates. Luciferase activity was measured 24-h post transfection by Dual Glo Luciferase Assay (Promega). Transfections were repeated in two independent experiments with similar results. The influence of the common and rare alleles of rs4407214 on promoter activity in the pGL3-Promoter vector (Invitrogen) were assessed using the same methodology. Primers are available on request. Electromobility shift assays Nuclear proteins from MCF10A and CAL51 cells were extracted using a hypotonic lysis buffer (10 mM HEPES, pH 7.9, 1.5 mM MgCl2, 10 mM KCL) supplemented with DTT and protease inhibitors, followed by an extraction buffer (20 mM HEPES, ph 7.9, 1.5 mM MgCl 2 , 0.42 M NaCl, 0.2 mM EDTA, 25% v/v glycerol) supplemented with DTT and protease inhibitors. Electrophoretic mobility shift assays probes were designed to cover each SNP ±20 base pairs, for both major and minor alleles. Probe pairs were dissolved in water and annealed at a concentration of 10 μM each. Probes were labelled with ATP (γ-32 P; Perkin Elmer) using T4 polynucleotide kinase and cleaned using the QiaQuick Nucleotide Removal Kit (Qiagen). Labelled and unlabelled probes were then incubated with protein extracts using LightShift Poly(dI–dC) (Thermo) and a binding buffer (10 mM Tris, 50 mM KCl, 1 mM DTT, pH 7.4) and electrophoresed on a 6% acrylamide gel overnight at 83 V. Gels were dried and films were exposed for 4–24 h. Probe sequences are shown in Supplementary Table 21 . How to cite this article : Couch, F. J. et al . Identification of four novel susceptibility loci for oestrogen receptor negative breast cancer. Nat. Commun. 7:11375 doi: 10.1038/ncomms11375 (2016).